Bright solid-state sources of indistinguishable single photons Bright sources of indistinguishable single photons are strongly needed for the scalability of quantum information processing. Semiconductor quantum dots are promising systems to build such sources. Several works demonstrated emission of indistinguishable photons while others proposed various approaches to efficiently collect them. Here we combine both properties and report on the fabrication of ultrabright sources of indistinguishable single photons, thanks to deterministic positioning of single quantum dots in well-designed pillar cavities. Brightness as high as 0.79±0.08 collected photon per pulse is demonstrated. The indistinguishability of the photons is investigated as a function of the source brightness and the excitation conditions. We show that a two-laser excitation scheme allows reducing the fluctuations of the quantum dot electrostatic environment under high pumping conditions. With this method, we obtain 82±10% indistinguishability for a brightness as large as 0.65±0.06 collected photon per pulse. The quantum interference [1] of two indistinguishable single photons is an important resource for long distance quantum communication and linear quantum computing [2] , [3] , [4] , [5] . Recent years have seen important progress in the development of bright single-photon sources in solid-state systems using semiconductor self-assembled quantum dots (QDs) [6] inserted in photonic structures [7] , [8] , [9] , [10] . QDs confine carriers in the three directions of space and present discrete energy states. When a laser pulse optically creates several electron-hole pairs in a QD, the system goes back to its ground state by emitting a cascade of photons. Thanks to the strong Coulomb interaction, only a single photon is emitted for a given emission energy [11] . This property has been exploited to generate single photons [6] , as well as single entangled photon pairs [12] , [13] . However, because only a few per cent of the emitted photons can be collected for QDs in bulk semiconductors, control of the QD spontaneous emission is needed to obtain bright quantum light sources. One can for instance insert the QD in a cavity to increase the local density of electromagnetic modes and accelerate its spontaneous emission into a given optical mode [14] , [7] , [8] , [10] . Another possibility is to use subwavelength waveguides to inhibit the emission in most directions of space [9] , [15] . State of the art extraction efficiencies around 40% in 0.4 numerical aperture have been reported with both geometries [8] , [9] , [10] . In nanowires, this extraction efficiency has been shown to reach 71±9% in a numerical aperture of 0.75 (ref. 9 ). Several works have also shown that single photons and entangled photon pairs can be made indistinguishable [16] , [17] , [18] . Shortening of the QD lifetime has been used to minimize the influence of dephasing processes and increase visibility [19] , [20] . However, combining high brightness and high indistinguishability is not straightforward. Indeed, to obtain high source brightness, a strong optical excitation of the quantum system is needed. Thus, many carriers are created in the QD environment, leading to dephasing, which is expected to reduce indistinguishability. In this article, we report on highly indistinguishable single-photon sources with unprecedented brightness obtained by deterministic [21] coupling of InGaAs QDs in pillars cavities. High indistinguishability is combined with high brightness thanks to a two colour excitation scheme. Extracting single photons with pillar microcavities When a QD is coupled to a cavity mode ( Fig. 1a ), its spontaneous emission into the cavity mode is accelerated by the Purcell factor F P (ref. 22 ). The fraction of photons emitted into the cavity mode is then given by β = F P /( F P +1) ( Fig. 1b ). The brightness of a source, defined by the number of collected photons in the first lens per excitation pulse, is given by the product βηq QD where η is the mode coupling to the external optical field and q QD the quantum efficiency of the QD emission line. Pillar cavities are obtained by etching a planar cavity made of two distributed Bragg reflectors around a λ microcavity [14] . We first note that absorption or scattering in the mirrors are negligible in the GaAs/AlAs system under consideration. Indeed, planar quality factors of a few 10 5 have been demonstrated using similar mirrors, only with a larger number of Bragg pairs [23] . To collect most photons from the top of the pillar, we use highly asymmetric cavities with a bottom mirror transmission more than three orders of magnitude smaller than the top mirror transmission. This strong unbalance in the mirror transmission ensures that less than 0.1% of photons escape through the bottom mirror [24] . However, losses can still arise from the sidewall roughness when reducing the pillar diameter. As a result, we expect the coupling to the external field to be given by η = Q / Q 0, where Q and Q 0 are the quality factors of the pillar mode and the planar cavity, respectively [25] . 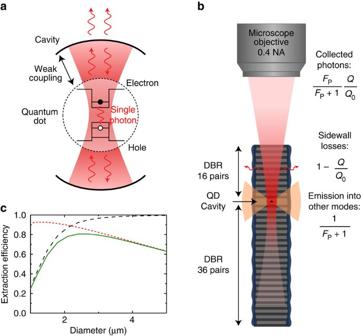Figure 1: Extracting single photons using Purcell effect in micropillar cavities (a) A semiconductor QD is inserted in a microcavity. (b) In micropillars, a fractionFP/(FP+1) of the photons is emitted into the cavity mode. Owing to losses at the sidewall roughness, only a fractionQ/Q0of these photons is collected in the first lens. (c) Fit of the experimentally measuredQ/Q0(black dashed line), calculatedFP/(FP+1) (red dotted line) and the maximum extraction efficiencyFP/(FP+1) ×Q/Q0(solid green line) as a function of micropillar diameters. Figure 1: Extracting single photons using Purcell effect in micropillar cavities ( a ) A semiconductor QD is inserted in a microcavity. ( b ) In micropillars, a fraction F P /( F P +1) of the photons is emitted into the cavity mode. Owing to losses at the sidewall roughness, only a fraction Q / Q 0 of these photons is collected in the first lens. ( c ) Fit of the experimentally measured Q / Q 0 (black dashed line), calculated F P /( F P + 1 ) (red dotted line) and the maximum extraction efficiency F P /( F P + 1 ) × Q / Q 0 (solid green line) as a function of micropillar diameters. Full size image Figure 1c shows a fit to typical experimentally measured Q / Q 0 for our etching conditions for a planar quality factor of Q 0 =3,000 (Methods). Q / Q 0 increases when increasing the pillar diameter and saturates close to 1 for a diameter around to 2 μm. Using this dependence for η and knowing the optical mode volume as a function of diameter, we can also predict the variation of β . Small diameters yield large Purcell factors and β, whereas large diameters lead to negligible losses due to sidewall roughness. Figure 1c shows that extraction efficiencies given by the product ηβ can be larger than 70% for diameters between 2 and 3 μm. However, to obtain such high brightness, the QD should be centred in the pillar and spectrally resonant with the cavity mode. Finally, InAs/GaAs self-assembled QDs have large overall quantum efficiencies (larger than 97%, see ref. 26 ). However, they have a non-negligible probability to be either in neutral, positively or a negatively charged exciton state under non-resonant optical pumping [27] . These charge state fluctuations would, therefore, reduce q QD and the source efficiency accordingly. As a result, QDs with a well-defined charged state should be selected. Obviously, gathering all these conditions is very demanding considering that QDs have random spectral and spatial positions. The absence of a deterministic technology to control the coupling between the QD and the cavity probably explains why such high brightnesses were not reported up to now. Bright single-photon sources Here we use the in situ lithography technique presented in ref. 21 to define pillar cavities centred on single selected QDs within 50 nm (Methods). The sources are fabricated from a planar cavity presenting a quality factor of Q 0 ≈3,000. As the mode energy depends on the pillar diameter, we selected QDs presenting the emission energies of pillar cavity modes with diameters between 2.5 and 3.5 μm. Finally, our technique provides the unique possibility to preselect QDs for which the emission of the neutral exciton emission is more than 10 times larger than the emission of both charged excitons. This ensures that q QD >0.9. The devices are characterized through micro-photoluminescence (PL) measurements at cryogenic temperatures. The sample is excited by a picosecond 82 MHz pulsed laser beam focused onto a 2-μm spot. The PL signal collected by the same objective is split in two paths and sent to spectrometers and detected with a liquid nitrogen cooled charge coupled device (CCD) or single-photon avalanche diodes (SPAD). The sample temperature is used to finely tune the spectral resonance between the cavity mode and the QD emission line [21] . The largest emission intensity is observed when the QD line is in perfect resonance with the cavity mode. 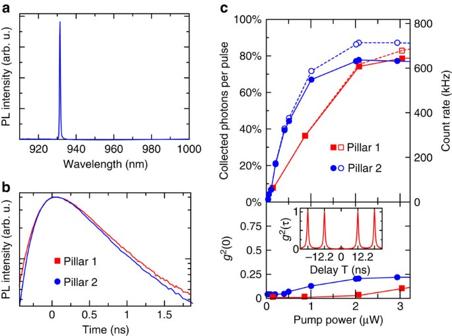Figure 2: Brightness of the single-photon source (a) PL spectrum of pillar 2 at spectral resonance with the cavity mode (10 K) and for an excitation power above the exciton line saturation. arb. u., arbitrary units. (b) PL intensity as a function of time for the exciton line in pillar 1 and 2. A lifetime around 265–270 ps is deduced after deconvolution with the temporal response of the system. Reference QDs in unprocessed planar cavity show decay time of 1.3 ns (not shown). (c) Top: Raw (open symbols) and multi-photon corrected (solid symbols) number of collected photons per laser pulse for pillar 1 (squares) and pillar 2 (circles). Bottom: Measuredg(2)(0) values as a function of the pump power. Inset: example of an antibunching curve measured at 2 μW for pillar 1. For all figures, the excitation laser is tuned to 860 nm to create carriers in the wetting layer. Resonance temperatures of the sources presented here are between 10 K and 21 K. Figure 2a presents the emission spectrum of pillar 2 with a pump laser tuned to 860 nm to create carriers in the wetting layer. At resonance between the exciton line and the cavity mode (10 K), only a single QD emission line is visible on a 90-nm wavelength spectral window. For this line, a 265±30 ps decay time is measured ( Fig. 2b ), corresponding to a Purcell factor of 3.9±0.6. A similar Purcell factor is measured for pillar 1, as shown in Fig. 2b . The count rate measured on one SPAD is presented in Fig. 2c as a function of incident power for both pillars. At saturation, the count rate is around 0.7 MHz. To deduce the corresponding number of photons collected per excitation pulse in the first lens, we calibrate all the optical components of the detection path ( Table 1 ). This count rate corresponds to a value as large as 0.9 photons collected per excitation pulse in the first lens. As recapture processes may affect this value by increasing the probability that more than one photon is emitted per excitation pulse, autocorrelation measurements are performed. We observe that the second order autocorrelation function at zero delay g (2) (0) is below 0.15 up to saturation so that the multi-photon correction term (1- g (2) (0)) 1/2 only slightly modifies the extremely high brightness ( Fig. 2c ). We thus obtain an experimentally measured brightness of 78±8%. Figure 2: Brightness of the single-photon source ( a ) PL spectrum of pillar 2 at spectral resonance with the cavity mode (10 K) and for an excitation power above the exciton line saturation. arb. u., arbitrary units. ( b ) PL intensity as a function of time for the exciton line in pillar 1 and 2. A lifetime around 265–270 ps is deduced after deconvolution with the temporal response of the system. Reference QDs in unprocessed planar cavity show decay time of 1.3 ns (not shown). ( c ) Top: Raw (open symbols) and multi-photon corrected (solid symbols) number of collected photons per laser pulse for pillar 1 (squares) and pillar 2 (circles). Bottom: Measured g (2) (0) values as a function of the pump power. Inset: example of an antibunching curve measured at 2 μW for pillar 1. For all figures, the excitation laser is tuned to 860 nm to create carriers in the wetting layer. Full size image Table 1 Experimental set-up calibration. Full size table Very high brightnesses ranging from 54±6% to 79±8% are measured on several pillar cavities in a 0.4 numerical aperture as shown in Table 2 . We also present the brightness of a QD line coupled to the mode of coupled pillars, a cavity which we recently used to collect entangled photon pairs [8] . For each source, we measure the lifetime of the QD transition and deduce the experimentally measured β = F P /( F P + 1 ) within a 10–20% error bar due to the finite time resolution of the photodiodes. While Q cannot be easily measured on the pillars embedding a single QD, we estimate that Q / Q 0 =0.95±0.05 from measurements on pillars embedding a high QD density. As shown in Table 2 , we observe a good agreement within error bars between the directly measured brightness and the measured expected value F P /( F P +1) × Q / Q 0 . Table 2 Experimental brightness of several sources. Full size table Indistinguishability and high brightness To prove the indistinguishability of two consecutively emitted photons, we implement the Hong Ou Mandel two-photon interference experiment [1] ( Fig. 3a ). The pillar 2 source is excited twice every laser pulse using a 2.2 ns delay line. Both emitted photons enter into a Michelson interferometer with a 2.2 ns delay between the two arms. Both photons exit the interferometer by the same output if they are Fourier-transform limited and present identical spatial mode, temporal profile, energy and polarization. Here the Purcell effect, implemented to collect the photons, also ensures that their spatial mode is the one of the cavity mode. Usually, polarization and energy properties are strongly related to the QD exciton transition. Indeed, because of anisotropy in the carrier wavefunctions, a single QD presents two exciton states with orthogonal linear polarizations. If this polarization splitting S is larger than the linewidth of the emission line, the photons emitted by the QD are indistinguishable only in the linear polarization basis corresponding to the QD axis [16] . Here we study annealed InGaAs QDs, similar to the one used to produce entangled photon pairs [8] . In this case, S is below 2 μeV so that Purcell effect leads to a radiative broadening of the exciton line overcoming the polarization splitting S. As a result, contrary to previous demonstrations [16] , [17] , [19] , we select any arbitrary linear polarization by inserting a polarizer before the interferometer. Finally, to reduce the effect of dephasing and obtain Fourier-transform limited photons, we take advantage of the Purcell effect to shorten the exciton lifetime [19] and investigate various excitation schemes. Note that the dephasing time of the emission lines measured as in ref. 7 does not relate to the photon indistinguishability measured using the Hong Ou Mandel experiment. Indeed, the latter measurement tests the indistinguishability of photons emitted 2.2 ns apart by the same QD. Longer time scale dephasing can broaden the emission line while not degrading the two-photon interference visibility. 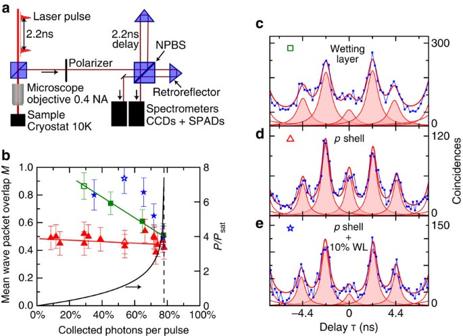Figure 3: Indistinguishability of the photons (pillar 2). (a) Experimental set-up used for indistinguishability measurements. (b) Mean wave packet overlap as a function of the number of collected photon per pulse for three excitation conditions. Square: pulsed excitation at 860 nm in the wetting layer. Triangle: pulsed excitation at 906 nm in thepshell of the QD. Stars: pulsed excitation in thepshell, with additional continuous wave excitation in the wetting layer contributing to 10% of the signal. Right scale: Excitation powerPnormalized to the saturation powerPsatas a function of the source brightness (solid black line). The dotted vertical line shows the maximum brightness of the source. Error in the evaluation ofMcomes from uncertainties in the fitting procedure of the various peak areas (see Methods). (c–e) Pulsed correlation histograms between the two SPADs for three excitation conditions indicated by the open symbols inFig. 3b. Experimental curves are blue symbols. Shaded curves are fit to the data with Lorentzian peaks. The measured mean wave packet overlap isM=86% forc,M=48% fordandM=92% fore. CCD, charge coupled device; NPBS, non polarizing beam splitter; WL, wetting layer. Figure 3: Indistinguishability of the photons (pillar 2). ( a ) Experimental set-up used for indistinguishability measurements. ( b ) Mean wave packet overlap as a function of the number of collected photon per pulse for three excitation conditions. Square: pulsed excitation at 860 nm in the wetting layer. Triangle: pulsed excitation at 906 nm in the p shell of the QD. Stars: pulsed excitation in the p shell, with additional continuous wave excitation in the wetting layer contributing to 10% of the signal. Right scale: Excitation power P normalized to the saturation power P sat as a function of the source brightness (solid black line). The dotted vertical line shows the maximum brightness of the source. Error in the evaluation of M comes from uncertainties in the fitting procedure of the various peak areas (see Methods). ( c–e ) Pulsed correlation histograms between the two SPADs for three excitation conditions indicated by the open symbols in Fig. 3b . Experimental curves are blue symbols. Shaded curves are fit to the data with Lorentzian peaks. The measured mean wave packet overlap is M =86% for c , M =48% for d and M =92% for e . CCD, charge coupled device; NPBS, non polarizing beam splitter; WL, wetting layer. Full size image We first study the indistinguishability under non-resonant excitation in the wetting layer at 860 nm. The Fig. 3c presents a correlation histogram of the interferometer two outputs at low excitation power. Peak at 0 delay corresponds to both photons entering the beam splitter simultaneously (the first photon follows the long arm of the interferometer and the second one the short arm). For a pure single-photon source with perfect indistinguishability, peak at 0 delay should vanish [1] . Deviation from this ideal situation arises from intrinsic properties of the sources, as well as imperfect instrumentation. Following ref. 16 to account for these various contributions (see Methods), we deduce a mean wave packet overlap M of 86±10%, a very high value for non-resonant excitation conditions. As shown in Fig. 3b , M decreases when increasing the excitation power, to reach 53±8% at maximum brightness of the source (green squares). The right scale shows the excitation power normalized to the saturation power P / P sat as a function of the source brightness given by I = βηq QD ( 1 - e - P / P sat ). Upon excitation power increase, the increasing number of carriers created in the wetting layer leads to fluctuations of the QD electrostatic environment and dephasing. To avoid this effect, resonant excitation in the p shell of the single QD state is used (906 nm). As shown in Fig. 3d , a lower wave packet overlap is obtained in this resonant excitation condition. A mean wave packet overlap around 50% is observed for all the excitation powers, up to saturation (red triangle in Fig. 3b ). The observation of such a low visibility under resonant excitation indicates that dephasing comes from fluctuations of the electrostatic environment around the QD. This observation is in contradiction with previous reports of high indistinguishabilities using p -shell resonant excitation [16] , [17] . Considering these two sets of measurements, we can conclude that under low power non-resonant excitation, non-resonantly created carriers fill deep traps around the QD and stabilize the QD electrostatic environment, enabling the observation of very high indistinguishability. Therefore, to obtain high indistinguishability combined with high brightness, we use p -shell strong excitation to saturate the QD transition while a second weak 860 nm continous wave excitation is applied to stabilize the QD electrostatic environment. Blue stars in Fig. 3b presents the corresponding experimental points where for each resonant excitation power, the second 860 nm laser produces 10% of the total intensity. The bottom scale then corresponds to the brightness due to the pulsed laser only. For all excitation powers up to 3 P sat , the two colour excitation scheme allows obtaining greatly improved indistinguishability as compared with single excitation schemes. For instance, the two colour experiment allows doubling the brightness as compared with a single colour scheme for a fixed mean wave packet overlap around 80%. A mean wave packet overlap of 92±11% is measured for a source brightness of 0.53±0.05 collected photons per pulse (Fig. 3e). This value remains as high as 82±10% for a brightness as large as 0.65±0.06 collected photon per pulse, corresponding to 2 P sat . Recent reports on QD spectroscopy have shown a strong instability of the QD charge state under strictly resonant excitation [28] , [29] , [30] , which could be overcome using a second non-resonant excitation with very low power. In the present measurement, the very high brightness of the source is observed either using wetting layer or p shell excitation, showing a very stable QD charge state. Here, the second laser helps minimizing fluctuations of carriers around the QDs, leading to a reduced dephasing and improved indistinguishability. To further increase both the source brightness and the photon indistinguishability, one could consider using the recently proposed adiabatic design of the cavity [31] , which makes the pillar mode less sensitive to the sidewall roughness. Using such a design, one could, therefore, further increase the Purcell factor hence β , while maintaining a good mode coupling to the external optical field. Stronger Purcell effect would also allow improving the indistinguishability by reducing the influence of fast dephasing [16] , [19] . Our work shows that ultrabright sources of single photons can be obtained thanks to a full control of the QD-pillar cavity system. High brightness and high indistinguishability can be combined thanks to an additional weak non-resonant excitation. Our results open the way to increasing the number of logic gates in optical quantum computers [3] thanks to the quantum statistics, high brightness and indistinguishability of QD-based sources. Sample fabrication The sample, grown by molecular been epitaxy, consists of a λ -cavity between two λ /4 n GaAs/Al 0.9 Ga 0.1 As Bragg reflectors with 16 (36) pairs for the top (bottom) mirror. A layer of InGaAs QDs is inserted in the cavity. The sample is annealed at 850 °C for 30 s to reduce the QD anisotropic polarization splitting. The in situ lithography technique is used to define pillars centred on single QDs [14] : a red laser beam is used to excite and monitor the QD emission so as to measure its spatial position with 50 nm accuracy. A green laser beam is used to expose a disk centred on the QD in a photoresist spin-coated on the sample. The in situ lithography was done using an attocube equipment (attoCFM for low temperature photolithography). Measuring the pillar Q factor To measure the planar cavity quality factor, we image the planar cavity mode dispersion and measure the cavity spectral linewidth at normal incidence. In Fig. 1c , the curve Q / Q 0 is a fit to measured Q factors on a sample with the same number of pairs in the mirrors but embedding a large QD density. Extraction efficiency measurements To measure the extraction efficiency of the source, all optical elements of the detection path have been calibrated using a continuous wave laser at 930 nm ( Table 1 ). The transmission of the spectrometer and the detection efficiency of the SPAD are estimated by measuring a pulsed laser signal of known power for which we can deduce the number of incident photons per pulse. Hanbury-Brown and Twiss interferometer The Hanbury-Brown and Twiss interferometer is composed of a 50/50 non-polarizing beam splitter (NPBS), which sends PL signals into (spectrometers coupled to SPADs). Indistinguability measurements To check the spatial overlap of the two photons in free space on the beam splitter, we take advantage of the source brightness to directly image the photon spatial modes on a liquid nitrogen cooled CCD. In the histograms presented in Fig 3c–e , Peak 0 (at 0 delay) corresponds to both photons entering the beam splitter simultaneously, peaks −1 (at -2.2 ns) and +1 (at 2.2 ns) correspond to the case where both photons take the same path. Peaks −2 (at -4.4 ns) and +2 (at 4.4 ns) correspond to first (second) photon following the short (long) arm. From obtained correlations histograms and from formulas, which give relative amplitude A −2 to A +2 of the five peaks in the centre of the histogram [16] , we deduce the value of the mean wave packet overlap M of two successive photons: R =0.476 and T =0.504 are reflection and transmission values of the beam splitter cube, ε =0.95 is the interference fringe contrast measured when monomode CW laser at 920 nm is sent into the interferometer. It accounts for optical surfaces imperfections. g is the autocorrelation function at zero delay g 2 (0), and the common prefactor N is related to the number of detected events. Error in the evaluation of M comes from uncertainties in the fitting procedure of the various peak areas and in the measurements of g and ε . The resulting error bars are displayed in Fig. 3b . How to cite this article: Gazzano O. et al. Bright solid-state sources of indistinguishable single photons. Nat. Commun. 4:1425 doi: 10.1038/ncomms2434 (2013).